The staphylococcal toxins γ-haemolysin AB and CB differentially target phagocytes by employing specific chemokine receptors Evasion of the host phagocyte response by Staphylococcus aureus is crucial to successful infection with the pathogen. γ-haemolysin AB and CB (HlgAB, HlgCB) are bicomponent pore-forming toxins present in almost all human S. aureus isolates. Cellular tropism and contribution of the toxins to S. aureus pathophysiology are poorly understood. Here we identify the chemokine receptors CXCR1, CXCR2 and CCR2 as targets for HlgAB, and the complement receptors C5aR and C5L2 as targets for HlgCB. The receptor expression patterns allow the toxins to efficiently and differentially target phagocytic cells. Murine neutrophils are resistant to HlgAB and HlgCB. CCR2 is the sole murine receptor orthologue compatible with γ-haemolysin. In a murine peritonitis model, HlgAB contributes to S. aureus bacteremia in a CCR2-dependent manner. HlgAB-mediated targeting of CCR2 + cells highlights the involvement of inflammatory macrophages during S. aureus infection. Functional quantification identifies HlgAB and HlgCB as major secreted staphylococcal leukocidins. S taphylococcus aureus is one of the most prominent causes of bacterial infections in humans worldwide [1] . S. aureus causes a plethora of infections, ranging from superficial skin infections to severe invasive diseases [2] . Emergence of methicillin-resistant S. aureus (MRSA) strains has become a global challenge for first-line antibiotic treatment regimens of infections with the pathogen [2] . Failure of vaccine development programmes poses an additional threat to public health and urges to a better understanding of the host–pathogen interaction [3] . A key host defence mechanism against S. aureus is the phagocyte-mediated killing [4] . The pathogen in return is well adapted to the human host, evading host immune responses at multiple levels using an arsenal of virulence factors [5] . A major mechanism deployed by S. aureus to target host phagocytes is the production of cytolytic toxins [6] . Staphylococcal leukocidins comprise a class of bicomponent pore-forming toxins capable of damaging the host cell plasma membrane [7] , [8] . The leukocidins characterized from human S. aureus isolates include Panton-Valentine Leukocidin LukSF (PVL) [9] , γ-haemolysin (HlgAB and HlgCB) [10] , [11] , LukED [12] and LukAB, also known as LukGH [13] , [14] . The genes encoding γ-haemolysin are present in over 99.5% of human S. aureus isolates. In contrast, carriage of the genes encoding other leukocidins such as PVL and LukED is not as widely distributed [15] , [16] . γ-haemolysin forms two functional bicomponent pore-forming toxins (HlgAB and HlgCB), which share the protein component HlgB [10] . In vitro , the expression of γ-haemolysin is highly upregulated during culture in blood [17] and during phagocytosis by neutrophils [6] . Some leukocidins exert cytotoxicity in a species-specific manner [18] , [19] . γ-haemolysin contributes partially to virulence during septic arthritis and systemic infection in mice [17] , [20] and endophthalmitis in rabbits [21] , [22] . However, to our knowledge, species-specific susceptibility of leukocytes to γ-haemolysin has never been investigated. Although the ganglioside GM1 was found to inhibit γ-haemolysin-dependent killing [23] , [24] , identification of the membrane glycolipid GM1 as a γ-haemolysin receptor cannot explain the observed cellular tropism of the toxins [7] . Cell selectivity and species specificity of PVL are determined by the interaction of PVL with the human complement receptors C5aR and C5L2 (ref. 18 ). In addition, LukED targets CCR5, CXCR1 and CXCR2 (refs 25 , 26 ). These receptors belong to the family of chemokine receptors, which play a crucial role in activation and migration of specific immune cells [27] , [28] . Here we report the identification of the human chemokine receptors CXCR1, CXCR2 and CCR2 as receptors for HlgAB and the human complement receptors C5aR and C5L2 as receptors for HlgCB. Toxin expression levels and functional pore-forming activity of different clinical S. aureus isolates underscore HlgAB and HlgCB as major secreted staphylococcal leukocidins. The abundant expression of the receptors on phagocytes makes them primary targets and allows the toxins to differentially discriminate phagocytic cells from other cells. We show that murine neutrophils are resistant to both HlgAB and HlgCB, and identify CCR2 as the sole murine receptor orthologue compatible with γ-haemolysin. Using a murine peritonitis model, we demonstrate that HlgAB contributes to S. aureus bacteremia in a CCR2-dependent manner. These findings highlight the involvement of inflammatory macrophages during S. aureus infection. γ-haemolysin AB and CB target chemokine receptors To evaluate the host target cell tropism of γ-haemolysin, we tested toxin-mediated cell permeability in freshly isolated human leukocytes using a membrane-impermeant fluorescent dye. 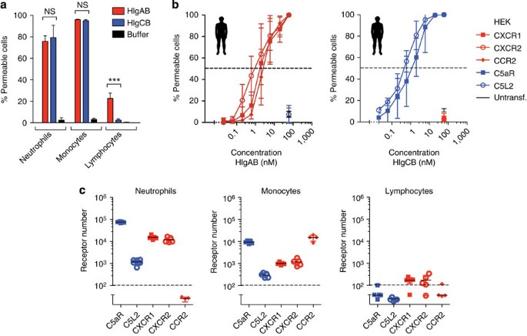Figure 1: HlgAB and HlgCB target human phagocytes expressing specific chemokine receptors. (a) HlgAB and HlgCB (63 nM) efficiently induce pore formation in human neutrophils and monocytes. HlgAB shows limited cytotoxicity towards lymphocytes. (b) Pore formation following treatment with HlgAB or HlgCB was monitored in HEK cells transfected with plasmids encoding human chemokine receptors. The dashed line indicates 50% pore formation. (c) Expression of chemokine receptors efficiently targeted by HlgAB and HlgCB was quantified on human leukocytes, showing abundant expression on phagocytes. The dashed line indicates the detection threshold. Permeable cells are propidium iodide or 4′,6-diamidino-2-phenylindole positive. Bars indicate s.d.,n=3–5. Statistical significance is displayed as ***P<0.005 using Student’st-test. See alsoSupplementary Fig. 1. Figure 1a confirms that HlgAB and HlgCB target human neutrophils and monocytes [29] . This pattern of cell specificity is similar to that of PVL [18] . In contrast to HlgCB, HlgAB shows limited cytotoxicity towards lymphocytes as well [30] . The extended cellular tropism of HlgAB compared with HlgCB implies the involvement of different host target cell receptors. Figure 1: HlgAB and HlgCB target human phagocytes expressing specific chemokine receptors. ( a ) HlgAB and HlgCB (63 nM) efficiently induce pore formation in human neutrophils and monocytes. HlgAB shows limited cytotoxicity towards lymphocytes. ( b ) Pore formation following treatment with HlgAB or HlgCB was monitored in HEK cells transfected with plasmids encoding human chemokine receptors. The dashed line indicates 50% pore formation. ( c ) Expression of chemokine receptors efficiently targeted by HlgAB and HlgCB was quantified on human leukocytes, showing abundant expression on phagocytes. The dashed line indicates the detection threshold. Permeable cells are propidium iodide or 4′,6-diamidino-2-phenylindole positive. Bars indicate s.d., n =3–5. Statistical significance is displayed as *** P <0.005 using Student’s t -test. See also Supplementary Fig. 1 . Full size image The molecular basis of cell selectivity of both HlgAB and HlgCB is not understood. Because PVL and HlgCB were predicted to share proteinaceous receptors [29] , we hypothesized that γ-haemolysin targets chemokine receptors as well. As no specific predictions were available for HlgAB, we screened human embryonic kidney (HEK) cells transfected with a collection of human chemokine receptors for cytotoxic susceptibility to HlgAB and HlgCB. Untransfected cells were resistant to pore formation induced by both HlgAB and HlgCB ( Fig. 1a,b ). Mirroring PVL specificity, HlgCB induced pore formation in cells transfected with the C5a receptors, C5aR or C5L2 ( Fig. 1b and Supplementary Fig. 6a ). In addition, HlgCB induced pore formation in cells transfected with the complement receptor C3aR, though only at high toxin concentrations ( Supplementary Fig. 1a ). Assessment of half-maximal effective lytic concentrations (EC 50 ) identified C5aR and C5L2 as the most efficient targets for HlgCB cytotoxicity, with ±100-fold lower EC 50 concentrations compared with C3aR ( Supplementary Fig. 1b ). HlgAB efficiently induced pore formation in cells transfected with the chemokine receptors CXCR1, CXCR2 and CCR2 ( Fig. 1b and Supplementary Fig. 6a ). Furthermore, high concentrations of HlgAB induced pore formation in cells overexpressing the chemokine receptor CXCR4 ( Supplementary Fig. 1a ). Calculation of EC 50 concentrations identified CXCR1, CXCR2 and CCR2 as the receptors most efficiently employed by HlgAB, with at least 30-fold lower EC 50 concentrations compared with CXCR4 ( Supplementary Fig. 1b ). Importantly, the respective panel of HlgAB and HlgCB receptors did not overlap ( Fig. 1b and Supplementary Fig. 1a ), indicating that HlgA and HlgC control receptor specificity. To obtain the affinity of the toxin–receptor interactions, surface plasmon resonance was performed using proteoliposomes containing C5aR, CXCR1, CXCR2 or CCR2. HlgC bound C5aR with a K D of 5.64 (±1.53) nM. HlgA bound CXCR1, CXCR2 and CCR2 with a K D of 5.69 (±1.94) nM, 27.20 (±5.54 nM) and 3.51 (±0.29) nM, respectively. Consistent with the cellular assays, no detectable binding of HlgC was observed on the HlgA receptors and vice versa ( Table 1 ). The restricted receptor spectrum emphasizes HlgAB and HlgCB as two different and specific toxins. Table 1 Apparent dissociation constants ( K D ) of HlgA and HlgC for chemokine receptors as determined by surface plasmon resonance analyses. Full size table In an attempt to better understand the leukocyte tropism of γ-haemolysin, we evaluated the expression levels of the receptors most efficiently employed by HlgAB and HlgCB on the surface of freshly isolated human leukocyte populations. The receptors targeted by HlgCB are present on neutrophils and monocytes, but absent on lymphocytes ( Fig. 1c ). These observations are in line with the cell specificity of HlgCB. The receptors employed by HlgAB are abundantly present on neutrophils and monocytes ( Fig. 1c ). CCR2 is exclusively expressed on monocytes. Low-level expression of CXCR1 and CXCR2 on lymphocytes likely accounts for the limited cytotoxicity of HlgAB towards these cells. In summary, these data suggest that the cellular tropism of γ-haemolysin is determined by the specific interaction of HlgA and HlgC with their respective protein receptors. The abundant expression of the efficient receptors on phagocytes allows the toxins to discriminate phagocytic cells from other cells. HlgAB and HlgCB lyse cells in a receptor-specific manner S. aureus isolates vary in both genetic contents and expression levels of leukocidins. Strain USA300 clone SF8300 is a minimally passed representative PVL-positive community-associated MRSA isolate from the United States [31] . S. aureus Newman is a PVL-negative, methicillin-sensitive strain frequently used for in vivo studies [32] . We tested the interaction of native HlgAB and HlgCB with specific receptors using bacterial culture supernatants. CXCR2-mediated cytotoxicity of HlgAB was confirmed using the supernatant of S. aureus USA300 SF8300 and its isogenic hlgACB mutant ( hlgACB knockout) strain [33] . Induction of pore formation in U937 promyelocytic cells stably transfected with CXCR2 was lost using supernatant of the strain lacking HlgACB. Pore-forming capacity of culture supernatant was restored by complementation with a plasmid encoding HlgAB, but not with a plasmid encoding HlgCB ( Fig. 2a and Supplementary Fig. 6b ). Due to the production of PVL, HlgCB cytotoxicity towards C5aR-transfected cells could not be investigated using a USA300 strain [18] . C5aR-mediated cytotoxicity of HlgCB was therefore validated using supernatants of strain Newman and its isogenic hlgACB mutant ( hlgACB knockout) strain [22] . Culture filtrates of Newman wild type but not of the strain lacking HlgACB were lytic to C5aR-transfected U937 cells. Cytotoxicity was restored by complementation with a plasmid encoding HlgCB, but not HlgAB ( Fig. 2b and Supplementary Fig. 6b ). 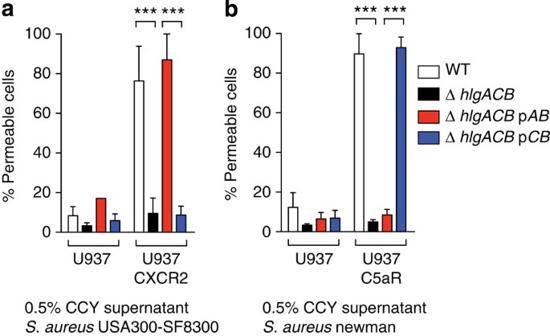Figure 2:S. aureus-secreted HlgAB and HlgCB lyse cells in a receptor-specific manner. Pore formation in transfected U937 cells was assessed following 30 min exposure to 0.5% bacterial culture supernatant (16 h culture in casein hydrolysate and yeast extract medium). (a) HlgAB in supernatant ofS. aureusstrain USA300 clone SF8300 induces CXCR2-specific lysis. (b) HlgCB in supernatant ofS. aureusstrain Newman induces C5aR-specific lysis. pAB:ΔhlgACBmutant complemented with a plasmid encodinghlgAB. pCB:ΔhlgACBmutant complemented with a plasmid encodinghlgCB. Permeable cells are propidium iodide PI or 4′,6-diamidino-2-phenylindole DAPI positive. Bars indicate s.d.,n=3–5. Statistical significance is displayed as ***P<0.005 using Student’st-test. Figure 2: S. aureus -secreted HlgAB and HlgCB lyse cells in a receptor-specific manner. Pore formation in transfected U937 cells was assessed following 30 min exposure to 0.5% bacterial culture supernatant (16 h culture in casein hydrolysate and yeast extract medium). ( a ) HlgAB in supernatant of S. aureus strain USA300 clone SF8300 induces CXCR2-specific lysis. ( b ) HlgCB in supernatant of S. aureus strain Newman induces C5aR-specific lysis. p AB : ΔhlgACB mutant complemented with a plasmid encoding hlgAB . p CB : ΔhlgACB mutant complemented with a plasmid encoding hlgCB . Permeable cells are propidium iodide PI or 4′,6-diamidino-2-phenylindole DAPI positive. Bars indicate s.d., n =3–5. Statistical significance is displayed as *** P <0.005 using Student’s t -test. Full size image These data confirm the results obtained with recombinant toxins, and demonstrate that HlgAB and HlgCB produced by S. aureus specifically target their respective host receptors. HlgAB and HlgCB are major secreted S. aureus leukocidins HlgCB shares receptors with PVL, while HlgAB partly shares receptors with LukED [18] , [25] , [26] . This finding suggests redundancy of the secreted toxins. To evaluate the relative importance of the different toxin–receptor pairs, we composed a panel of representative European clinical S. aureus strains isolated from blood cultures. As most of European S. aureus strains are PVL negative [16] , we included the PVL-positive major MRSA clone currently causing infections in the United States (USA300 LAC) as a control [34] . All the selected European clinical isolates were methicillin susceptible, and belonged to a variety of clonal complexes ( Table 2 ). Table 2 HlgAB and HlgCB are major secreted S. aureus leukocidins. Full size table We first determined which genes encoding secreted leukocidins are present in the different clinical isolates. Confirming expectations [7] , [15] , [16] , all clinical strains contained the genes encoding hlgA and hlgC , while none contained the lukS-PV gene. Following clonal lineage [35] , half of the isolates encoded the lukE gene ( Table 2 ). Next, we evaluated the expression of the leukocidin S-component mRNAs by quantitative reverse transcriptase-PCR. For PVL, culture broth-dependent differential expression of the toxin has been described [17] , [36] , [37] . Strain USA300 LAC confirmed this broth-dependent expression of lukS-PV ( Supplementary Fig. 2 a,b ). Quantities of lukE transcripts were broth dependent as well. In contrast, all clinical strains consistently expressed high levels of hlgA and hlgC mRNA in the two different culture broths tested ( Table 2 and Supplementary Fig. 2a,b ). To investigate the relative contribution to pore formation of the respective secreted leukocidins, we subsequently tested supernatants of the different bacterial cultures on human neutrophils and HEK cells stably transfected with specific receptors. Untransfected HEK cells showed background pore formation of ±15% on average ( Supplementary Fig. 2b–d,f,g ). Culture supernatants of all clinical isolates efficiently induced pore formation in HEK cells transfected with C5aR or CCR2 ( Table 2 and Supplementary Figs 2b,d, 6c ), indicating that HlgCB and HlgAB are secreted in functional quantities. Although HEK cells transfected with CCR5 showed susceptibility to recombinant LukED as expected ( Supplementary Figs 2e, 6c ) [25] , pore formation by culture supernatants in CCR5-expressing HEK cells was inefficient and not linked to lukE expression ( Table 2 and Supplementary Fig. 2 a,b,f ). However, culture supernatants of the clinical isolates induced efficient pore formation in HEK cells transfected with CXCR1 ( Supplementary Figs 2c, 6c ). As CCR5-expressing HEK cells remained largely unaffected by the culture supernatants, it is likely that HlgAB mainly drives cytotoxicity towards CXCR1-transfected cells. Similar to cells expressing CCR5, pore formation in HEK cells co-transfected with CD11b/CD18 (CR3) was inefficient ( Supplementary Figs 2g, 6c ). All culture supernatants showed high cytotoxic activity towards human neutrophils, which abundantly express the γ-haemolysin receptors C5aR, CXCR1 and CXCR2 ( Fig. 1c , Table 2 and Supplementary Fig. 2h ). Altogether, near-universal prevalence and consistent toxin expression discriminate γ-haemolysin from other staphylococcal leukocidins, and identify HlgAB and HlgCB as highly significant secreted S. aureus toxins efficiently targeting phagocytic cells. HlgAB and HlgCB induce proinflammatory responses In addition to inducing pore formation, staphylococcal leukocidins have proinflammatory properties [33] , [38] , [39] . Sublytic concentrations of PVL prime neutrophil responses in a C5aR-dependent manner [18] . We thus tested if immune activating properties of HlgAB and HlgCB were receptor mediated. HlgCB and HlgAB at low concentrations increased the N -formyl-methionine-leucine-phenylalanine (fMLP)-induced oxidative burst by neutrophils in a similar way as tumour necrosis factor α, C5a and interleukin-8 (IL-8, CXCL8). Priming by HlgCB was fully antagonized after preincubation of cells with the specific C5aR-antagonist CHIPS 31–121 ( Fig. 3a and Supplementary Fig. 3a ) [40] . This finding demonstrates that the C5aR drives priming of neutrophils by sublytic concentrations of HlgCB. To our knowledge, no molecules are available that antagonize both human CXCR1 and CXCR2. Therefore, we tested the CXCR2-specific proteolytic enzyme Staphopain-A for interference with HlgAB [41] . As expected based on the presence of CXCR1, preincubation of cells with Staphopain-A alone did not affect priming by HlgAB ( Fig. 3b and Supplementary Fig. 3b ). 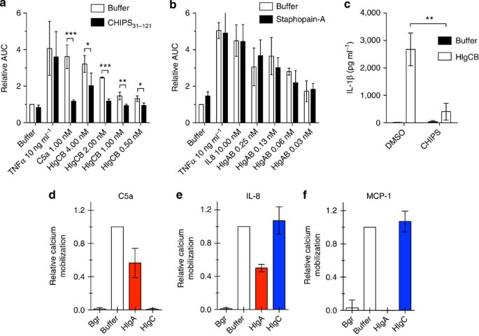Figure 3: HlgAB and HlgCB induce proinflammatory responses, and single components HlgA and HlgC are immunomodulatory molecules. (a,b) Oxidative burst of human neutrophils induced by 1 μM fMLP after priming with 10 ng ml−1tumour necrosis factor α (TNFα), 1 nM C5a, 10 nM IL-8 and (a) 0.50 to 4.00 nM HlgCB or (b) 0.03 to 0.25 nM HlgAB. Cells were pretreated with (a) 700 nM of the specific C5aR antagonist CHIPS31–121or (b) 500 nM of the CXCR2-specific proteolytic enzyme Staphopain-A. Oxidative burst, detected by luminescence, is expressed as relative area under the curve (AUC). (c) IL-1β production in the supernatant of primary human monocyte-derived macrophages intoxicated with 20.00 nM HlgCB. Cells were pretreated with 700 nM CHIPS or dimethyl sulphoxide (DMSO). (d–f) Calcium mobilization with (d) 0.1 nM C5a, (e) 0.5 nM IL-8 in human neutrophils and (f) 1.0 nM MCP-1 in human monocytes inhibited by 94.0 nM HlgA or HlgC. Bars indicate s.d.,n=3–4. Statistical significance is displayed as *P<0.05; **P<0.01 and ***P<0.005 using Student’st-test. Figure 3: HlgAB and HlgCB induce proinflammatory responses, and single components HlgA and HlgC are immunomodulatory molecules. ( a , b ) Oxidative burst of human neutrophils induced by 1 μM fMLP after priming with 10 ng ml −1 tumour necrosis factor α (TNFα), 1 nM C5a, 10 nM IL-8 and ( a ) 0.50 to 4.00 nM HlgCB or ( b ) 0.03 to 0.25 nM HlgAB. Cells were pretreated with ( a ) 700 nM of the specific C5aR antagonist CHIPS 31–121 or ( b ) 500 nM of the CXCR2-specific proteolytic enzyme Staphopain-A. Oxidative burst, detected by luminescence, is expressed as relative area under the curve (AUC). ( c ) IL-1β production in the supernatant of primary human monocyte-derived macrophages intoxicated with 20.00 nM HlgCB. Cells were pretreated with 700 nM CHIPS or dimethyl sulphoxide (DMSO). ( d – f ) Calcium mobilization with ( d ) 0.1 nM C5a, ( e ) 0.5 nM IL-8 in human neutrophils and ( f ) 1.0 nM MCP-1 in human monocytes inhibited by 94.0 nM HlgA or HlgC. Bars indicate s.d., n =3–4. Statistical significance is displayed as * P <0.05; ** P <0.01 and *** P <0.005 using Student’s t -test. Full size image In human macrophages, HlgCB activates inflammasome signalling [33] . CHIPS, a specific C5aR antagonist [42] , antagonized IL-1β release induced by HlgCB ( Fig. 3c ). This finding implies that the C5aR mediates the release of proinflammatory cytokine IL-1β in response to HlgCB. Taken together, these findings indicate that the C5aR mediates the proinflammatory properties of HlgCB. CXCR1 and CXCR2 likely mediate priming of neutrophils by HlgAB. HlgA and HlgC are immunomodulatory molecules Following activation with their natural ligands, signal transducing chemokine receptors provoke transient rises of intracellular calcium. Low concentrations of the single-protein components HlgA and HlgC are not activating or cytotoxic [43] . Since both proteins bind chemokine receptors, we tested if HlgA and HlgC act as functional antagonists of the respective receptors by detection of intracellular calcium mobilization. As HlgC binds the signal transducing C5aR, we tested if HlgC acts as a functional inhibitor of this receptor. Just as LukS-PV, HlgC antagonized activation induced by C5a on neutrophils ( Fig. 3d ) [18] . Because C5L2 is an atypical chemokine receptor and not coupled to a G-protein [44] , the functional inhibition of this receptor by HlgC could not be tested. HlgA interacts with CXCR1, CXCR2 and CCR2. HlgA antagonized the activation of neutrophils induced by IL-8 (a ligand of both CXCR1 and CXCR2; Fig. 3e ) [45] . In addition, HlgA inhibited activation of monocytes induced by the CCR2-specific ligand MCP-1 (CCL2; Fig. 3f ). These data suggest that the binding proteins of γ-haemolysin as single components have receptor-specific immunomodulatory properties. HlgAB and HlgCB feature receptor selectivity in mice S. aureus interacts with the host immune system in a highly human-specific manner [5] . To explore murine susceptibility to γ-haemolysin, we tested the cytotoxicity of HlgAB and HlgCB towards murine bone marrow-derived leukocytes. As observed for PVL, murine neutrophils and monocytes were resistant to HlgCB-induced pore formation ( Fig. 4a ). In line with this result, HEK cells transfected with the murine C5aR or C5L2 were resistant to HlgCB ( Fig. 4b and Supplementary Fig. 6d ). 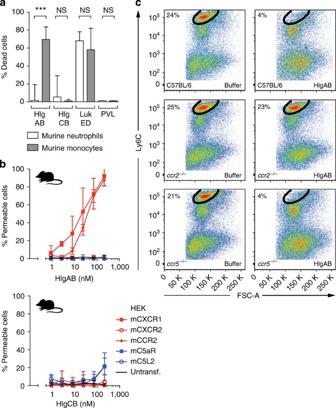Figure 4: Murine phagocytes display selective sensitivity and resistance to HlgAB and HlgCB. (a) Pore formation in murine bone marrow-derived neutrophils (CD11b+, Ly6G+) and monocytes (CD11b+, Ly6G−, Ly6Chigh) following incubation with leukocidins (190 nM) identifies murine monocytes as the sole murine phagocytes susceptible to γ-haemolysin. Dead cells are fixable viability dye positive. (b) Pore formation by HlgAB and HlgCB of HEK cells transfected with plasmids encoding murine chemokine receptors confirms susceptibility and resistance of primary murine phagocytes. Permeable cells are propidium iodide or 4′,6-diamidino-2-phenylindole positive. (c) Depletion of murine bone marrow-derived monocytes (CD11b+, Ly6G−, Ly6Chigh) by HlgAB (12,5 nM) is CCR2-dependent as shown as concatenates of three individual mice in each group of C75BL/6 wild type,ccr2−/−andccr5−/−mice. Bars indicate s.d.,n=3. Statistical significance is displayed as ***P<0.005 using Student’st-test. See alsoSupplementary Fig. 4. Figure 4: Murine phagocytes display selective sensitivity and resistance to HlgAB and HlgCB. ( a ) Pore formation in murine bone marrow-derived neutrophils (CD11b + , Ly6G + ) and monocytes (CD11b + , Ly6G − , Ly6C high ) following incubation with leukocidins (190 nM) identifies murine monocytes as the sole murine phagocytes susceptible to γ-haemolysin. Dead cells are fixable viability dye positive. ( b ) Pore formation by HlgAB and HlgCB of HEK cells transfected with plasmids encoding murine chemokine receptors confirms susceptibility and resistance of primary murine phagocytes. Permeable cells are propidium iodide or 4′,6-diamidino-2-phenylindole positive. ( c ) Depletion of murine bone marrow-derived monocytes (CD11b + , Ly6G − , Ly6C high ) by HlgAB (12,5 nM) is CCR2-dependent as shown as concatenates of three individual mice in each group of C75BL/6 wild type, ccr2 −/− and ccr5 −/− mice. Bars indicate s.d., n =3. Statistical significance is displayed as *** P <0.005 using Student’s t -test. See also Supplementary Fig. 4 . Full size image HlgAB and LukED both target human CXCR1 and CXCR2 ( Fig. 1b ) [26] . However, murine neutrophils were resistant to HlgAB-induced pore formation ( Fig. 4a ). In mice, CXCR2, but not CXCR1, is expressed on neutrophils and monocytes [46] . Although HEK cells transfected with murine CXCR1 were susceptible to HlgAB-induced cytotoxicity, cells transfected with murine CXCR2 remained unaffected by HlgAB ( Fig. 4b and Supplementary Fig. 6d ). The incompatibility of HlgAB with murine CXCR2 explains resistance of murine neutrophils to the toxin. In contrast, LukED is compatible with murine CXCR2 ( Supplementary Fig. 4a ), accounting for susceptibility of murine neutrophils towards LukED ( Fig. 4a ). Monocytes of wild-type and ccr5 −/− mice were susceptible to HlgAB-induced pore formation, whereas monocytes of ccr2 −/− mice were HlgAB resistant ( Fig. 4a,c ). In agreement with this, HEK cells transfected with the murine CCR2 showed clear sensitivity to HlgAB ( Fig. 4b and Supplementary Fig. 6d ). Murine bone marrow cells from ccr2 −/− mice did not release IL-1β when exposed to HlgAB, in constrast to cells from wild-type mice ( Supplementary Fig. 4b ). These results provide further evidence for a specific interaction of HlgAB with CCR2. Collectively, our data show that γ-haemolysin features distinct receptor-mediated specificity in mice and human. As a consequence, murine neutrophils are resistant to both HlgAB and HlgCB. Importantly, the results identify HlgAB and CCR2 as potential subjects for investigation in murine models of staphylococcal infection. HlgAB targeting of CCR2 enhances S. aureus pathogenesis Although the genes encoding γ-haemolysin are present in nearly all human S. aureus isolates, its contribution to staphylococcal pathophysiology is not fully understood. Since we discovered that HlgAB targets CCR2, we investigated the contribution of this interaction to S. aureus pathogenesis in vivo in a murine peritonitis model. Inflammatory macrophages in the peritoneal cavity of mice, elicited by heat-inactivated S. aureus , express CCR2 ( Fig. 5a ) [47] . 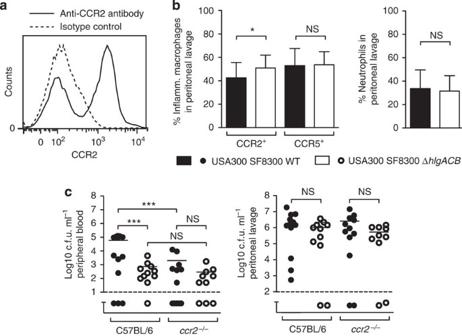Figure 5: HlgAB targeting of CCR2 contributes toS. aureuspathogenesis. (a) Murine peritoneal inflammatory macrophages (CD11b+, Ly6G−, F4/80+) elicited by heat-inactivatedS. aureusexpress CCR2. Concatenates are shown, withn=2–3. (b) Mice intraperitoneally infected with wild-typeS. aureusstrain USA300 clone SF8300 show relatively less CCR2+but equal CCR5+peritoneal inflammatory macrophages compared withΔhlgACBbacteria infected mice at 24 h post infection. Mice infected with wild-type orΔhlgACBbacteria have similar proportions of neutrophils (CD11b+, Ly6G+) in the peritoneal cavity. (c) C57BL/6 wild-type mice intraperitoneally infected withΔhlgACBbacteria show lower amounts of bacteria in the peripheral blood at 24 h post infection than mice infected with wild-type bacteria.ccr2−/−mice infected with wild-type bacteria show lower amounts of bacteria in the peripheral blood at 24 h post infection than C57BL/6 wild-type mice, independently ofhlgACB. All mice show similar amounts of bacteria in the peritoneal lavage fluid. Bars express mean with s.d., withn=10–15 per group of mice distributed over at least two independent experiments. Dashed lines indicate detection thresholds. Statistical significance is displayed as *P<0.05 and ***P<0.005 using Student’st-test or two-way analysis of variance with Bonferroni post-test correction for multiple comparison where appropriate. See alsoSupplementary Fig. 5. Figure 5: HlgAB targeting of CCR2 contributes to S. aureus pathogenesis. ( a ) Murine peritoneal inflammatory macrophages (CD11b + , Ly6G − , F4/80 + ) elicited by heat-inactivated S. aureus express CCR2. Concatenates are shown, with n =2–3. ( b ) Mice intraperitoneally infected with wild-type S. aureus strain USA300 clone SF8300 show relatively less CCR2 + but equal CCR5 + peritoneal inflammatory macrophages compared with ΔhlgACB bacteria infected mice at 24 h post infection. Mice infected with wild-type or ΔhlgACB bacteria have similar proportions of neutrophils (CD11b + , Ly6G + ) in the peritoneal cavity. ( c ) C57BL/6 wild-type mice intraperitoneally infected with ΔhlgACB bacteria show lower amounts of bacteria in the peripheral blood at 24 h post infection than mice infected with wild-type bacteria. ccr2 −/− mice infected with wild-type bacteria show lower amounts of bacteria in the peripheral blood at 24 h post infection than C57BL/6 wild-type mice, independently of hlgACB . All mice show similar amounts of bacteria in the peritoneal lavage fluid. Bars express mean with s.d., with n =10–15 per group of mice distributed over at least two independent experiments. Dashed lines indicate detection thresholds. Statistical significance is displayed as * P <0.05 and *** P <0.005 using Student’s t -test or two-way analysis of variance with Bonferroni post-test correction for multiple comparison where appropriate. See also Supplementary Fig. 5 . Full size image To investigate the γ-haemolysin-mediated targeting of CCR2, we monitored the presence of CCR2 + inflammatory macrophages in the peritoneal cavity of mice infected with S. aureus USA300 clone SF8300 or its isogenic hlgACB mutant ( hlgACB knockout) strain [33] , [48] . Mice infected with wild-type S. aureus showed a significant decrease in the proportion of CCR2 + inflammatory macrophages compared to mice infected with the hlgACB mutant strain ( Fig. 5b ). Notably, in the same mice, the fraction of CCR5 + macrophages was equal between wild-type- and hlgACB mutant-infected mice. In agreement with the resistance of murine neutrophils to γ-haemolysin, mice infected with wild-type and hlgACB mutant had similar proportions of neutrophils ( Fig. 5b ). Using another USA300 clone, LAC [34] , and its isogenic hlgA mutant strain ( hlgA::bursa ), the observed modulation of the CCR2 + inflammatory macrophage population was shown to be HlgA specific ( Supplementary Fig. 5a ). These data demonstrate that during infection HlgAB is active and specifically targets CCR2 + inflammatory macrophages in the peritoneal cavity. Staphylococcal peritonitis is used as a model to study the spread of bacteria into the bloodstream [49] . We observed that the number of viable bacteria in the peripheral blood of mice is dependent on the presence of both HlgAB and CCR2. Twenty four hours after intraperitoneal infection, wild-type mice infected with S. aureus USA300 clone SF8300 had ±100-fold higher counts of viable bacteria in the peripheral blood compared with wild-type mice infected with the hlgACB mutant strain ( Fig. 5c ). Using USA300 clone LAC and its isogenic hlgA mutant, the bacteremia was confirmed to be driven specifically by HlgA ( Supplementary Fig. 5b ). Cellular recruitment in response to sterile inflammatory stimuli is impaired in ccr2 −/− mice [50] . In contrast, infection with S. aureus induced similar influx of macrophages into the peritoneal cavity of wild-type and ccr2 −/− mice ( Supplementary Fig. 5c ). Compared with wild-type mice, infection of ccr2 −/− mice with S. aureus USA300 clone SF8300 resulted in ±100-fold lower numbers of bacteria in the peripheral blood ( Fig. 5c ). The number of bacterial counts in the peripheral blood of ccr2 −/− mice was independent of γ-haemolysin. Moreover, no statistically significant differences were observed in the bacterial counts of the peritoneal cavity after 24 h in all infected mice ( Fig. 5c and Supplementary Fig. 5b ), representing comparable levels of bacteria as the seeding source. These results demonstrate that HlgAB contributes to S. aureus bacteremia in a CCR2-dependent manner. In addition, the interaction of HlgAB with CCR2 + cells highlights the involvement of inflammatory macrophages during S. aureus infection. γ-haemolysin is highly prevalent in human S. aureus isolates [15] , [16] . Strikingly, its contribution to pathophysiology is poorly understood. As clinical epidemiology is inadequate in the context of high prevalence, a functional approach is needed to assess the role of γ-haemolysin in staphylococcal virulence. We show that HlgAB and HlgCB use chemokine receptors to induce pore formation in the target cell membrane. Comparison of half-maximal effective concentrations needed to induce specific pore formation allows the discrimination between efficient and inefficient receptors. While HlgAB efficiently targets CXCR1, CXCR2 and CCR2, the other toxin combination HlgCB efficiently targets C5aR and C5L2. Affinities of HlgA and HlgC for the respective receptors are in nanomolar range, a finding that is consistent with other leukocidins and their proteinaceous receptors [25] , [51] , [52] . On the basis of studies with LukED [26] , it is likely that different domains of the toxins dictate receptor selectivity. The staphylococcal leukocidins HlgAB, HlgCB, PVL and LukED share considerable homology. LukAB however, is distinctive and more distantly related [53] . This divergence might account for the interaction of HlgAB, HlgCB, PVL and LukED with chemokine receptors, while LukAB strictly targets the CD11b subunit of the integrin Mac1 (ref. 52 ). The previously proposed cellular association of γ-haemolysin with the ganglioside GM1 alone [23] , [24] failed to explain cell type specificities of the toxins [7] . Expression levels of the involved chemokine receptors on human leukocytes contribute to a better understanding of the cellular tropism of the toxins [30] . The abundant expression of the efficient receptors on phagocytes makes them major targets and allows the toxins to discriminate phagocytic cells from other cells. In addition to cytotoxic capacities, HlgAB and HlgCB have proinflammatory and immunomodulatory properties as well. Just as for PVL, our data support the notion that both HlgAB and HlgCB engage the respective chemokine receptors directly and specifically during priming and inflammasome activation [7] , [18] . Simultaneous expression and secretion of the toxins as bicomponents—as observed here—however allows immediate formation of cytolytic pores on the target cells. Although the binding of HlgA and HlgC to the receptors results in antagonism of neutrophil and monocyte activation in vitro , it remains unclear if functional inhibition by single-protein components contributes to pathogenesis of S. aureus . The impact of γ-haemolysin on the virulence of S. aureus is incompletely understood. We suspect this is in part due to adaptation of S. aureus to the human host [5] . Indeed, our results show that current mouse models are not suitable to investigate the interaction of γ-haemolysin with C5aR, C5L2, CXCR1 and CXCR2. As a result, γ-haemolysin cytotoxicity towards neutrophils cannot be addressed in mice. Another consequence is that the apparent redundancy of LukED versus HlgAB, and PVL versus HlgCB cannot be studied in vivo currently. Since immunogenic resemblance limits the development of specific monoclonal antibodies for detection of leukocidin subunits, we developed an alternative approach to investigate the relative contribution to pore formation of the different leukocidins. Using cell lines expressing specific chemokine receptors and culture supernatants of a panel of diverse clinical S. aureus isolates, we demonstrate that HlgAB and HlgCB are functionally major secreted staphylococcal leukocidins employing phagocyte specific chemokine receptors. Since the clinical isolates tested were PVL negative, the cytotoxicity towards C5aR-transfected cells is likely due to high expression of HlgCB as observed with mutant strains. As all clinical isolates show potent cytotoxic activity towards CCR2-transfected but not CCR5-transfected cells, the expression and secretion of HlgAB most probably mediates CXCR1-specific toxicity as indicated with experiments using mutant strains. We demonstrate that the expression and secretion of γ-haemolysin AB and CB by various clinical S. aureus isolates in different conditions are consistent and functionally highly effective when compared with other members of the family of staphylococcal bicomponent pore-forming toxins. These observations are in line with reports investigating the expression during culture in blood and after phagocytosis [6] , [17] , and indicate that HlgAB and HlgCB are prominent secreted toxins engaging receptors abundantly expressed on phagocytic cells. The high expression of both HlgCB and HlgAB allows the pathogen to differentially target phagocytes. The interaction of HlgAB with CCR2, a chemokine receptor most notably expressed on monocytes and inflammatory macrophages, is exclusive and non-redundant in relation to other staphylococcal leukocidins [18] , [25] , [26] , [52] . CCR2 is the only compatible murine γ-haemolysin receptor orthologue. Using a murine peritonitis model, we validated the specific interaction of HlgAB with CCR2. S. aureus decreases the proportion of CCR2 + inflammatory macrophages in a HlgAB-dependent manner. In addition, we identified HlgAB as a virulence factor contributing to bacteremia by employing its host counterpart, CCR2. Importantly, the numbers of macrophages in the infected peritoneal cavity of wild-type and ccr2 −/− mice were similar. Furthermore, hlgACB mutant bacteremia levels were not statistically significant between wild-type and ccr2 −/− mice. While we cannot exclude a contribution of CCL2/CCR2 signalling [54] , [55] , these observations strongly suggest that the reported phenotype in wild-type versus ccr2 −/− mice is due to a specific targeting of CCR2 by HlgAB and not due to a broad immune defect of ccr2 −/− mice. Interestingly, a previous study described a mild impact on virulence of γ-haemolysin in a murine intravenous infection model [17] . This contribution likely reflects the interaction between HlgAB and CCR2. Future research is needed to provide detailed insights into the mechanisms involved in controlling bacteremia by HlgAB-mediated targeting of CCR2 + cells in the peritoneal cavity. The genes encoding γ-haemolysin are present in nearly all human S. aureus isolates. The other leukocidin encoded by all S. aureus strains, LukAB, was previously reported to bind the bacterial surface and to promote survival by facilitating bacterial escape after phagocytosis [13] , [14] , [56] . Thus, LukAB has been proposed to act from within the phagocyte [56] . Pore formation induced by the different culture supernatants tested in HEK cells co-transfected with CD11b/CD18 was incomplete, indeed suggesting that the toxin is inefficiently secreted into the supernatant. In contrast, quantification of the expression levels and pore-forming capacity of all tested clinical S. aureus isolates identify HlgAB and HlgCB as highly significant secreted S. aureus toxins efficiently targeting phagocytic cells. Altogether, these data highlight the differential and complementary mechanisms that S. aureus deploys to target phagocytes. Ethics statement Human leukocytes were isolated after informed consent was obtained from all subjects in accordance with the Declaration of Helsinki. Approval was obtained from the medical ethics committee of the UMC Utrecht, The Netherlands. All experiments involving animals were reviewed and approved by the animal ethics committees of Lyon, France (CECCAPP, protocol number ENS2012_033). Recombinant protein production and purification S. aureus strains used to amplify coding sequences of toxins are shown in Supplementary Table 1 . HlgA, HlgB, HlgC, LukE, LukD, LukS-PV and LukF-PV were cloned and expressed as described elsewhere [33] . Briefly, the coding sequences omitting the regions predicted to encode the signal peptide were cloned and transformed into E. coli M15 or BL21 pLys. The protein expression was induced by adding isopropyl-β- D -thiogalactopyranoside during exponential growth of transformed E. coli . Polyhistidine-tagged proteins were isolated from supernatants of cell lysates on Ni-nitrilotriacetic acid columns (Qiagen). Contaminating lipopolysaccharide was eliminated using a Polymixin-B column (Thermo Scientific). Bacterial strains and culture S. aureus strains used for this study are listed in Table 2 and Supplementary Table 2 . Complementation of Δ hlgACB mutants and generation of an erythromycin sensitive USA300 LAC Δ hlgA strain is described in Supplementary Methods . Clinical S. aureus strains, isolated from blood cultures with a diverse infection focus and originating from patients admitted to the intensive care unit of the University Medical Center Utrecht, The Netherlands, were randomly chosen from a database created for tertiary hospital routine diagnostics. Standard microbiological diagnostic techniques were applied for microbial identification and antibiotic resistance profiling. All strains were cultured in casein hydrolysate and yeast extract [36] , [37] or brain heart infusion, and overnight supernatants filter sterilized. For in vivo experiments, mid-exponential subcultures were washed extensively in PBS. Typing of clinical S. aureus isolates All clinical S. aureus isolates used in this study were typed by multi-locus sequence typing [57] . Using the eBURST algorithm, isolates were assigned to a clonal complex [58] . Leukocidin S-component PCRs were performed on genomic DNA, which was isolated as previously described [42] . Primers were designed to be highly gene specific ( Supplementary Table 3 ). S. aureus RNA extraction and cDNA synthesis S. aureus RNA was isolated from samples using an RNeasy Plus Mini Kit (Qiagen) following the manufacturer’s instructions. Bacteria were precultured overnight and subsequently diluted in fresh medium for culture to early stationary phase (6.5 h; OD 660 ±1.5). Bacteria were spun for 30 s at 13,000 r.p.m. Pellets were briefly kept in liquid nitrogen to stop bacterial metabolism, and resuspended in buffer RLT containing β-mercaptoethanol (Sigma). Resuspended bacteria were added to silica beads (Merlin), and disrupted using a mini-Beadbeater (BioSpec Products) for 1 min at 3,500 r.p.m. After cooling of the samples for 1 min on ice, an additional two cycles of disruption were applied. Contaminating chromosomal DNA was removed by consecutive treatment of samples with RNAse Free DNAse (Qiagen) and a RapidOut DNA Removal Kit (Thermo Scientific). RNA yield was measured using a NanoDrop ND1000 (NanoDrop Technologies), and quality was checked on agarose gel. Contamination with genomic DNA was excluded by a PCR specific for genomic DNA. Standardized quantities of total RNA were used immediately for synthesis of cDNA with a Maxima First Strand cDNA Synthesis Kit for RT-qPCR (Thermo Scientific). Quantitative real-time PCR cDNA from the equivalent of 10 ng mRNA was used to perform qPCR for hlgA , hlgC , lukE and lukS-PV using SYBR Green Master Mix (Qiagen) in a 7300 Real Time PCR System (Applied Biosystems) according to the manufacturer’s instructions. cDNA from the equivalent of 1 ng mRNA was used to amplify 16S as an endogenous control. Primers used to detect specific transcripts are listed in Supplementary Table 4 . These primers are based on toxin sequences from strains Newman and USA300 ( lukS-PV ). Triplicate reactions for each primer set containing approximately 100 copies of S. aureus USA300 clone LAC genomic DNA were included to calibrate transcript abundance of each toxin. C T values were collected over 40 cycles of PCR, with primer annealing at 60 °C, and data collection during the 30 s extension step at 72 °C. Analysis was performed using 7300 Real-Time PCR System Software. Relative transcript abundance was calculated by the comparative C T (ΔΔ C T ) method, using 16S as the endogenous control and USA300 clone LAC genomic DNA as the calibrator sample. Samples with an average C T value greater than 32 were considered background and were excluded from analysis. Toxin expression is indicated as the log 10 of the fold change in relative transcript abundance of each toxin compared with abundance from amplification from USA300 clone LAC genomic DNA. Cell isolations Human leukocytes, obtained from healthy volunteers, were isolated by Ficoll/Histopaque centrifugation [42] . Bone marrow of mice was harvested and immune cells collected as described [18] . Mice receiving intraperitoneal injections with heat-inactivated S. aureus USA300 SF8300 Δ hlgACB (1 × 10 8 c.f.u., at 0 and 24 h) were killed after 48 h. Immune cells were collected by peritoneal lavage with PBS. All in vitro experiments with cells were performed with RPMI (Invitrogen) supplemented with 0.05% human serum albumin (Sanquin) unless specified otherwise, with cell concentrations adjusted to 5 × 10 6 cells ml −1 . Quantification of human leukocyte receptor expression levels Freshly isolated human leukocytes were incubated in a total volume of 50 μl at 5 × 10 6 cells ml −1 on ice with 10 μg ml −1 mouse anti-human chemokine receptor monoclonal antibodies for C5aR (clone S5/1, AbD SeroTec), C5L2 (clone 1D9-M12, Bio Legend), CXCR1 (clone 42705, R&D), CXCR2 (clone 48311, R&D) and CCR2 (clone 48607, R&D), followed by fluorescein isothiocyanate-conjugated goat-anti-mouse antibody (1:50, Dako). Antibody binding was quantified by calibration to defined antibody binding capacity units using QIFIKIT (Dako) and corrected for isotype controls. Cell lines and transfections U937 cells (a promyelocytic cell line) stably transfected with C5aR, CXCR2 or an empty expression vector were obtained from Eric R. Prossnitz (University of New Mexico, Albuquerque, NM, USA) [59] . Human C5aR, C5L2, C3aR, CXCR1, CXCR2, CCR1, CCR2 and CCR5 and murine C5aR, C5L2, CXCR1, CXCR2, and CCR2 were cloned into a pcDNA3.1 vector (Invitrogen) as described previously [18] . All genes reside on a single exon. Amplification reactions were performed on QUICK-Clone cDNA of human bone marrow or mouse liver (BD Biosciences Clontech) using PfuTurbo DNA polymerase (Stratagene). Plasmids encoding human C5L2 and CXCR2 were purchased from the UMR cDNA Resource Center. Plasmids encoding CXCR3, CXCR4 and CXCR6 were purchased from Thermo Fisher. Primer designs, restriction sites and accession numbers used in this study are displayed in Supplementary Table 5 . HEK293T cells (a HEK cell line) were transiently transfected according to the manufacturer’s protocols with 4 μg DNA and 5 μl Lipofectamine 2000 (Life Technologies) [18] . After 24 h, transfected cells were harvested with 0.05% Trypsin/0.53 mM EDTA. Maximal pore formation of HEK293T cells transiently transfected with plasmids encoding chemokine receptors was defined by the percentage of receptor expressing cells as independently determined by flow cytometry. For the construction of HEK293T cells stably expressing human C5aR, CXCR1, CCR2, CCR5 or CR3 (CD11b/CD18), we cloned the complete coding regions of these receptors ( Supplementary Table 6 ) into the bicistronic expression plasmid pIRESpuro3 (Clontech). CD18 was cloned into pIRESpuro3, whereas CD11b was cloned into pIREShyg3 (Clontech). For stable expression, the constructs were transfected into HEK293T cells using Lipofectamine 2000 (Life Technologies). One day after transfection, cells were put under selection pressure using 1 μg ml −1 puromycin in Dulbecco's modified Eagle’s medium with 10% fetal calf serum. A few weeks later, cells were subcloned and tested for stable receptor expression by flow cytometry. The expression of human chemokine receptors on transfected cells was defined using 10 μg ml −1 mouse anti-human chemokine receptor monoclonal antibodies for C5aR (clone S5/1, AbD SeroTec), C5L2 (clone 1D9-M12, Bio Legend), C3aR (clone 534625, R&D), CXCR1 (clone 42705, R&D), CXCR2 (clone 48311, R&D), CXCR3 (clone 49801, R&D), CXCR4 (clone 12G5, R&D), CXCR6 (clone MAB699, R&D), CCR1 (clone 53504, R&D), CCR2 (clone 48607, R&D) and CCR5 (clone 2D7, BD), followed by PE-labelled goat anti-mouse antibody (1:80, DAKO). For cells expressing CR3, cells were stained with an APC-labelled mouse monoclonal antibody directed towards CD18 (clone L130, 1:50, BD) and a fluorescein isothiocyanate-labelled mouse monoclonal antibody detecting CD11b (clone ICRF44, 1:10, BD). Receptor expression levels were similar within each panel of transfected cells for all receptors ( Supplementary Fig. 6a–c ). As no monoclonal antibodies are available for all involved murine chemokine receptors, the expression of murine receptors was defined by co-transfection with an internal ribosome entry site-green fluorescent protein encoding pCDNA3 vector (Invitrogen) [60] . Green fluorescent protein expression was similar for all murine receptors investigated, and fully correlated with susceptibility of cells transfected with toxin-compatible receptors ( Supplementary Fig. 6d ). Cell permeability assays Cells were exposed to recombinant proteins or overnight bacterial culture supernatant in a volume of 50–100 μl. Human peripheral blood mononucleated cell were prestained for CD14 expression (clone M5E2, 1:10, BD). Cells were incubated with toxin for 30 min at 37 °C. Human leukocytes and cell lines were subsequently analysed by flow cytometry and pore formation was defined as intracellular staining by propidium iodide (PI) or 4′,6-diamidino-2-phenylindole. After treatment with Fcγ-receptor block, murine cell surfaces were stained with antibodies directed towards CD11b (clone M1/70, 1:400, BD), Ly6G (clone 1A8, 1:100, BD), Ly6C (clone AL-21, 1:200, BD) and F4/80 (clone BM8, 1:600, Bio Legend) antibodies. Following exposure to toxins, murine cells were incubated on ice with the fixable viability dye eFluor 780 (1:1,000, eBiosciences) and cell viability was subsequently analysed by flow cytometry in the presence of Flow-Count Fluorospheres (BD). Cell viability was defined as eFluor 780 negative cells in relation to buffer-treated cells. Analysis of pore formation in transiently transfected HEK293T cells was limited to receptor-positive cells. Half-maximal effective lytic concentrations were calculated using nonlinear regression analyses. As leukocidins are two-component toxins, equimolar concentrations of polyhistidine-tagged proteins were used. To minimize bias due to the production of the nonspecifically cytotoxic phenol-soluble modulins, experiments with culture supernatants were performed in the presence of 10% fetal calf serum [61] , [62] . Surface plasmon resonance studies Surface Plasmon Resonance of HlgA and HlgC and chemokine receptor proteoliposomes was performed using the Biacore T100 system and the series S L1 sensor chip using 10 mM Tris 1 mM MgCl 2 and 1 mM CaCl 2 as the running buffer. Wheat-germ proteoliposomes of CXCR1, CXCR2, CCR2 and C5aR (Abnova) at a final protein concentration of 20 μg ml −1 were immobilized onto test flow cells with a flow rate of 10 μl min −1 for 10 min with a minimum capture level of 600RU. Empty, mock wheat-germ proteoliposomes (Abnova) were immobilized onto the reference flow cell using the same conditions with a minimum capture level of 300RU being obtained. Single-cycle kinetics was initially used to establish concentration ranges for HlgA and HlgC for each chemokine receptor liposome with concentrations ranging from 0.01 to 20 μg ml −1 with 5 μg ml −1 used as the maximum concentration used in multiple cycle kinetics. A flow rate of 30 μl min −1 was used for analysis with a contact time of 1 min and a disassociation time of 10 min for each concentration used. To ensure that the chemokine receptors captured on the L1 chip were biologically relevant, MCP-1 (Peprotech) was tested against CCR2. Concentrations between 16 and 500 ng ml −1 were tested. The affinity of MCP-1 with the captured CCR2 liposome was found to be 0.84±014 nM on three replicate experiments. This was within the reported values found in the literature indicating that the proteoliposomes were in their native conformation [63] . Neutrophil priming Priming of human neutrophils has been described in detail recently [18] . Briefly, neutrophils were incubated for 5 min with 700 nM CHIPS 31–121 to block the C5aR, or for 15 min with 500 nM Staphopain-A to cleave the amino-terminal CXCR2. Cells were primed with 10 ng ml −1 TNFα, 1 nM C5a, 10 nM IL-8 or a range of sublytic concentrations of HlgCB or HlgAB for 30 min at 37 °C. Subsequently, chemiluminescence was recorded in a luminometer. After 30 s of baseline recording, a final concentration of 1 μM fMLP was injected to stimulate the oxidative burst. For each sample, the area under the curve after addition of fMLP was calculated. For comparison of experiments, area under the curve values were expressed relative to buffer-treated cells stimulated with fMLP. IL-1β production Derivation of primary human macrophages from monocytes is described elsewhere [33] . To induce pro-IL-1β and prime the NLRP3-inflammasome, human macrophages were treated with heat-killed S. aureus at a multiplicity of 100:1 for 16 h [33] . Cells were washed twice to remove heat-killed S. aureus and exposed to toxin during 1 h at 37 °C. Murine bone marrow cells were pretreated with 250 ng ml −1 lipopolysaccharide for 3 h and subsequently intoxicated with 6 nM HlgAB or 20 μM Nigericin during 30 min at 37 °C. Release of human and murine IL-1β into the supernatant was quantified by enzyme linked immunosorbent assays (DuoSet ELISA kits, R&D Systems) [33] . Calcium mobilization assays Activation of human neutrophils and monocytes was performed by real-time detection of calcium mobilization using flow cytometry [18] . Human monocytes were labelled with an anti-CD14 monoclonal antibody (BD). Cells, labelled with Fluo-3AM, were preincubated with HlgA or HlgC for 1 min at room temperature. Subsequently, baseline fluorescence was recorded in a flow cytometer. After 10 s of baseline recording, C5a (Sigma), IL-8 or MCP-1 (PeproTech) was added and fluorescence was recorded for an additional 50 s. Relative increase in fluorescence was expressed in comparison to uninhibited cells. Murine in vivo experiments C57BL/6 wild-type mice were obtained from Charles River Laboratories. ccr2 −/− and ccr5 −/− mice (Jackson Laboratories) were bred in house. Eight to 9-week-old age- and sex-matched mice were infected intraperitoneally with 0.5 ml PBS containing 1 × 10 8 c.f.u. of bacteria. At 24 h post infection, peripheral blood was obtained and mice were killed to recover peritoneal lavage fluid. Peripheral blood and peritoneal lavage fluid were plated to evaluate the bacterial burden. After incubation on ice with the fixable viability dye eFluor 780, peritoneal cells were treated with Fcγ-receptor block and stained with monoclonal antibodies detecting CD11b, Ly6G, Ly6C, F4/80 and CCR2 (clone 475301, 1:100, R&D) or CCR5 (clone HMCCR5, 1:100, Bio Legend). Cells were subsequently analysed by flow cytometry and viable cells were defined as eFluor 780 negative cells. In the model of staphylococcal peritonitis, mortality of mice was equal for all groups (±20%). Graphical and statistical analyses Flow cytometric analyses were performed with FlowJo (Tree Star Software). Statistical analyses were performed with Prism (GraphPad Software). Statistical significance was calculated using analysis of variance and Student’s t -tests where appropriate. How to cite this article: Spaan, A. N. et al. The staphylococcal toxins γ-haemolysin AB and CB differentially target phagocytes by employing specific chemokine receptors. Nat. Commun. 5:5438 doi: 10.1038/ncomms6438 (2014).